Large modulation of zero-dimensional electronic states in quantum dots by electric-double-layer gating Electrical manipulation and read-out of quantum states in zero-dimensional nanostructures by nano-gap metal electrodes is expected to bring about innovation in quantum information processing. However, electrical tunability of the quantum states in zero-dimensional nanostructures is limited by the screening of gate electric fields. Here we demonstrate a new way to realize wide-range electrical modulation of quantum states of single self-assembled InAs quantum dots (QDs) with a liquid-gated electric-double-layer (EDL) transistor geometry. The efficiency of EDL gating is 6–90 times higher than that of the conventional solid gating. The quantized energy level spacing is modulated from ~15 to ~25 meV, and the electron g -factor is electrically tuned over a wide range. Such a field effect tuning can be explained by the modulation in the confinement potential of electrons in the QDs. The EDL gating on the QDs also provides potential compatibility with optical manipulation of single-electron charge/spin states. Following Moore’s law, top-down nanofabrication technology has tremendously driven the scaling of device sizes of Si metal–oxide–semiconductor (MOS) transistors. With this technological trend extrapolated, the device miniaturization will soon meet its physical limits [1] . Therefore, the use of bottom-up nanostructures as an active channel of transistors becomes increasingly important and attracts considerable attention for their prospective applications, especially to quantum information processing [2] , [3] , [4] , [5] , [6] . One of the promising techniques for electrical access to extremely small bottom-up nanostructures is the use of nano-gap metal electrodes [7] , [8] , [9] , [10] , [11] . Electron tunnelling through single self-assembled InAs quantum dots (QDs) coupled to nano-gap metal electrodes has been intensively investigated. To date, a variety of remarkable properties of the InAs QD transistors has already been revealed, such as artificial-atom properties [11] , [12] , electrically tunable large g -factors [13] and spin–orbit interaction [5] , [14] , [15] , and optical pumping of carriers in the terahertz frequency range [6] . However, electrical tuning of the electronic states in the QDs over a wide range has so far been elusive and remains as a great challenge. Electric-double-layer (EDL) transistors with ionic liquids as gate dielectric have recently emerged as a powerful tool in tuning the Fermi energy, E F , in solids [16] , [17] , [18] , [19] , [20] , [21] , [22] , [23] , [24] , [25] . The EDL formed at liquid/solid interfaces functions as nano-gap capacitors with a huge capacitance and can accumulate or deplete charge carriers over a wide range. Although the EDL gating technique has so far been applied only to two- and one-dimensional (2D and 1D) electron/hole systems [16] , [17] , [18] , [19] , [20] , [21] , [22] , [23] , [24] , [25] , the EDL gating of zero-dimensional (0D) QDs is not reported yet but is of great interest because tremendous gating power of EDL allows us to widely modulate electronic states in ultrasmall 0D QDs, providing us with a key to develop novel device concepts and also to broaden the novel applications of 0D bottom-up nanostructures. In this article, by EDL gating with an ionic liquid, we demonstrate large electrical modulation of electronic states including the electron-charging energy, level quantization energy and even Lande g -factor in single InAs QDs. QD electric-double-layer transistor Transport measurements were performed on a single InAs self-assembled QD contacted with nano-gap source-drain electrodes, as shown in Fig. 1c . To tune the electronic states of the InAs QDs, we fabricated a double-gate structure; the EDL gate was used to accumulate or deplete charge carrier over a wide range, whereas the back-gate electrode was used for the fine tuning of the energy levels in the QD ( Fig. 1a ). Figure 2a shows the transfer characteristics (source-drain current, I SD , as a function of the EDL-gate voltage, V EDL ) of an InAs EDL transistor measured at 215 K. The device shows a typical n-type accumulation operation with a small hysteresis, which is caused by charge trapping probably by the surrounding QDs (see Fig. 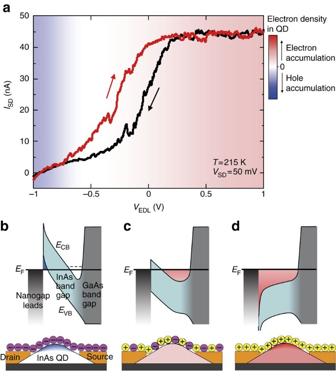Figure 2: Transport properties measured at 215 K. (a) Transfer characteristics (ISD−VEDL) of an InAs QD transistor with an EDL gate measured at 215 K. The transfer characteristics of each sample were reproducible and the curves of three consecutive scans were almost overlapped with each other. (b–d) Schematic energy band diagrams (upper panel) and carrier distributions in the InAs QDs (lower panel) atVEDL~−1 V (b),~0 V (c) and ~1 V (d). The conduction and the valence bands are denoted asECBandEVB, respectively. 1c ). With an increase in V EDL in the positive direction, cations accumulate right above the InAs QD and induce electrons in the QD, as shown in Fig. 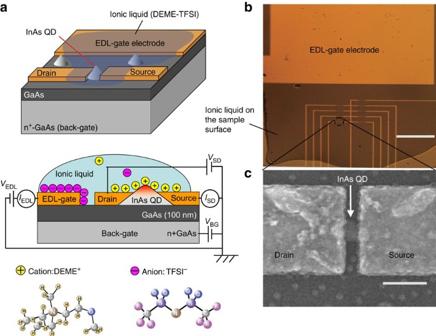1a . Figure 1: Quantum dot electric-double-layer transistor. (a) Schematic diagrams of the liquid-gated EDL transistor based on a single InAs QD. The cations and anions are DEME+and TFSI−, respectively. (b) An optical microscope image of a fabricated sample showing the nano-gap metal electrodes and the EDL-gate electrodes immersed in the optically transparent ionic liquid (DEME-TFSI). Scale bar, 50 μm. (c) A scanning electron microscope image of the nano-gap metal electrodes bridged by a single InAs QD. The metallurgical size of the InAs QD used in this study was about 70 nm × 110 nm × 25 nm. Scale bar, 150 nm. Figure 1: Quantum dot electric-double-layer transistor. ( a ) Schematic diagrams of the liquid-gated EDL transistor based on a single InAs QD. The cations and anions are DEME + and TFSI − , respectively. ( b ) An optical microscope image of a fabricated sample showing the nano-gap metal electrodes and the EDL-gate electrodes immersed in the optically transparent ionic liquid (DEME-TFSI). Scale bar, 50 μm. ( c ) A scanning electron microscope image of the nano-gap metal electrodes bridged by a single InAs QD. The metallurgical size of the InAs QD used in this study was about 70 nm × 110 nm × 25 nm. Scale bar, 150 nm. Full size image Figure 2: Transport properties measured at 215 K. ( a ) Transfer characteristics ( I SD − V EDL ) of an InAs QD transistor with an EDL gate measured at 215 K. The transfer characteristics of each sample were reproducible and the curves of three consecutive scans were almost overlapped with each other. ( b – d ) Schematic energy band diagrams (upper panel) and carrier distributions in the InAs QDs (lower panel) at V EDL ~−1 V ( b ),~0 V ( c ) and ~1 V ( d ). The conduction and the valence bands are denoted as E CB and E VB , respectively. Full size image In Fig. 2a , one can see that the conductance of the sample starts to increase and saturates at V EDL >0.2 V. This current saturation is likely caused by the screening of the gate electric field by electrons accumulated near the top of the InAs QD, as schematically illustrated in Fig. 2d . Once a large number of electrons are accumulated, the electronic states in the QD do not change in the region where the metal electrodes can probe, resulting in the observed saturation in I SD at V EDL >0.2 V. Note that such kind of current saturation behaviour has never been observed before in the conventional solid-gated QD systems and implies that an extremely high electric field strength is induced by the EDL gating. When the InAs QD is negatively biased, the electron number in the InAs QD decreases, which results in the reduction in I SD . The decrease in I SD continues until InAs QD becomes depleted. More detailed discussion based on the data measured at lower temperatures will be made later. 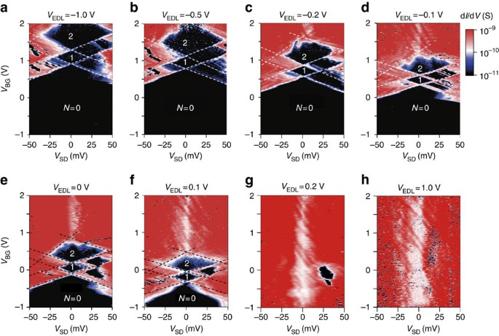Figure 3: Low-temperature transport properties at various EDL-gate voltages. (a–h) Coulomb stability diagrams measured at 3.5 K forVEDL=−1 V (a), −0.5 V (b), −0.2 V (c), −0.1 V (d), 0 V (e), 0.1 V (f), 0.2 V (g) and 1.0 V (h). These Coulomb stability diagrams were measured while sweepingVEDLto the negative direction (black curve inFig. 2a). The asymmetric shape of the Coulomb diamond is because of the asymmetric tunnel coupling between the QD and the source/drain electrodes. The dashed lines are guides for eyes. Large modulation of electronic states in QDs Figure 3a–h shows the Coulomb stability diagrams obtained by measuring the differential conductance, d I /d V SD , as a function of the source-drain voltage, V SD , and the back-gate voltage, V BG , at 3.5 K for various V EDL (see Supplementary Note 1 and Supplementary Figs S1–S3 for the universality of this phenomenon). Diamond-like patterns (Coulomb diamonds) that reflect single-electron tunnelling can be seen in Fig. 3a–f , and the Coulomb diamonds for electron number N =1 and 2 are clearly resolved (for details, see Supplementary Figs S4 and S5 ). Although the Coulomb diamonds for N ≥3 are not clearly observed in this QD sample, EDL gating effects on the electronic structures of the InAs QD can be discussed by using the N =1 and 2 Coulomb diamonds. In Fig. 3a–f , the Coulomb diamond for N =2 is notably larger than that for N =1, which is attributed to the shell structure in the InAs QD [11] , [12] . Figure 3: Low-temperature transport properties at various EDL-gate voltages. ( a – h ) Coulomb stability diagrams measured at 3.5 K for V EDL =−1 V ( a ), −0.5 V ( b ), −0.2 V ( c ), −0.1 V ( d ), 0 V ( e ), 0.1 V ( f ), 0.2 V ( g ) and 1.0 V ( h ). These Coulomb stability diagrams were measured while sweeping V EDL to the negative direction (black curve in Fig. 2a ). The asymmetric shape of the Coulomb diamond is because of the asymmetric tunnel coupling between the QD and the source/drain electrodes. The dashed lines are guides for eyes. 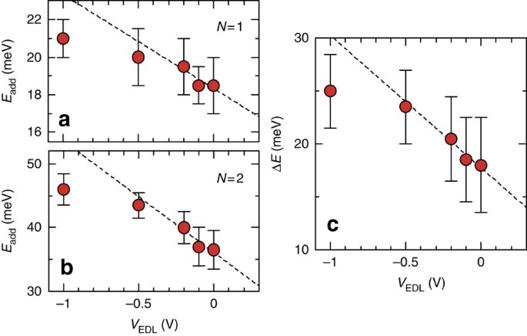Figure 4: EDL-gate voltage dependence of the electronic states in the QD. Charge addition energy,Eadd, forN=1 (a) and 2 (b) as a function ofVEDLdetermined from the Coulomb stability diagrams inFig. 3(see alsoSupplementary Figs S4 and S5). (c) Difference in the charge addition energies betweenN=1 and 2, ΔE=Eadd(N=2)−Eadd(N=1), as a function ofVEDL. When the charge addition energy was polarity-dependent, which is the case seen inFig. 3a–f, the size of the Coulomb diamonds was determined as the average values of the two. The dashed lines are guides for eyes. The error bars originate from broad edges of the Coulomb diamonds inFig. 3because of strong tunnel coupling between the metal source-drain electrodes and the electrons in the QD. Full size image Figure 4a,b shows the charge addition energy at N , E add ( N ), as a function of V EDL , plotted for N =1 and 2, respectively. E add (1), which corresponds to the charging energy of the ground state, monotonically increases from 18 to 21 meV with decreasing V EDL . This result indicates that the electron wave function for the ground state shrinks with decreasing V EDL , leading to smaller capacitive coupling with the electrodes and enhanced electron–electron Coulomb repulsion in the QD. In the constant-interaction model, the difference in E add between N =1 and 2, Δ E , corresponds to the difference in the quantization energy between the ground and the first excited states [26] . In Fig. 4c , Δ E is plotted as a function of V EDL , from which one can see that Δ E monotonically increases from ~15 to ~25 meV with decreasing V EDL . Using the simple square potential well approximation, the effective lateral confinement sizes at V EDL =−1 and 0.1 V are roughly estimated to be ~50 and~70 nm, respectively, which are in reasonable agreement with our previous report on the QD size dependence of Δ E [12] . It should be noted that we are able to electrically modulate the electron orbital states in a QD continuously by the EDL gating. So far, the field effect by the EDL gating has been discussed only in terms of the rigid-band shift approximation [16] , [17] , [18] , [19] , [20] , [21] , [22] , [23] , [24] , [25] . Although our results cannot be interpreted with the rigid-band model, it is able to be well-interpreted in terms of the modulation in the shape of confinement potential of electrons in the QD. Figure 4: EDL-gate voltage dependence of the electronic states in the QD. Charge addition energy, E add , for N =1 ( a ) and 2 ( b ) as a function of V EDL determined from the Coulomb stability diagrams in Fig. 3 (see also Supplementary Figs S4 and S5 ). ( c ) Difference in the charge addition energies between N =1 and 2, Δ E = E add ( N =2)− E add ( N =1), as a function of V EDL . When the charge addition energy was polarity-dependent, which is the case seen in Fig. 3a–f , the size of the Coulomb diamonds was determined as the average values of the two. The dashed lines are guides for eyes. The error bars originate from broad edges of the Coulomb diamonds in Fig. 3 because of strong tunnel coupling between the metal source-drain electrodes and the electrons in the QD. Full size image Modulation of electron g -factor Next, let us look into how the EDL gating affects the electron spin properties of InAs QDs. 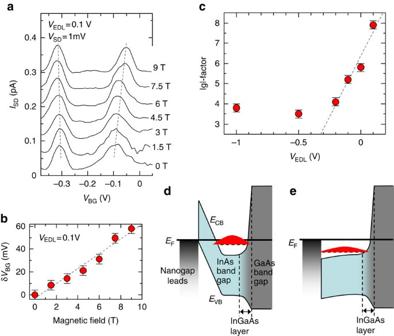Figure 5: Electrong-factor for various EDL-gate voltages. (a) The first and the second Coulomb oscillation peaks measured at various magnetic fields whenVEDL=0.1 V. Magnetic fields were applied perpendicular to the substrate. The curves are offset by 0.05 pA. (b) Magnetic field variation of theVBGspacing between the first and the second Coulomb peaks. The error bars come from the uncertainties in the Coulomb peak positions because of current noise. (c) Electrong-factors of the ground state for variousVEDL. The error bars arise from errors both in the linear fit of the data inFig. 5b(dashed line) and in the back-gate lever-arm factors (seeSupplementary Fig. S6). (d) Schematic energy band diagram of the QD sample with negativeVEDL(approximately −0.5 V). The conduction and the valence bands of the InAs surface are pushed up and, as a result, InAs surface is depleted. (e) Energy band diagram with positiveVEDL(~0.1 V). The surface energy band is bent down and the surface depletion layer vanishes, resulting in a larger confinement size of electrons. The dashed lines are guides for eyes. Figure 5a shows the first and second Coulomb oscillation peaks measured at various magnetic fields, B , when V EDL =0.1 V. Clear peak shift is observed with increasing B -field because of the presence of both the diamagnetic shift and the Zeeman effect. Figure 5b shows the B -field variation of the V BG spacing between the first and the second Coulomb peaks, δ V BG . The δ V BG increases linearly with increasing B -field, indicating the lifting of the spin degeneracy of the ground states because of Zeeman splitting. From this splitting, the electron g -factor for the ground state can be derived to be | g |~7.9. In the same manner, the electron g -factor can be determined at various V EDL and plotted in Fig. 5c (for details, see Supplementary Figs S6 and S7 ). As seen in the figure, it is found that the electron g -factor strongly depends on V EDL and increases with increasing V EDL . The electrical tuning of electron g -factor in InAs QDs has been reported so far [13] , [27] , [28] , [29] . The electron g -factor in InAs QDs is strongly influenced by the quantum confinement effect and alloy composition in the QDs [13] . It is known that, in self-assembled InAs QDs grown at ~500 °C, a large composition gradient from GaAs to InAs is formed up to 3–5 nm above the GaAs/InAs interface because of the In–Ga intermixing effect [12] , [30] , [31] . As shown in Fig. 5d , when V EDL <−0.5 V, the surface of the InAs QD is depleted and a large portion of the electron wave function resides in the Ga-rich layer around the bottom of the QD, leading to a small g -factor that reflects the small g -factor in GaAs (| g GaAs |=0.44). On the other hand, when V EDL ~0.1 V, a larger portion of the electron wave function extends in the In-rich region as shown in Fig. 5e , resulting in a larger g -factor. Figure 5: Electron g -factor for various EDL-gate voltages. ( a ) The first and the second Coulomb oscillation peaks measured at various magnetic fields when V EDL =0.1 V. Magnetic fields were applied perpendicular to the substrate. The curves are offset by 0.05 pA. ( b ) Magnetic field variation of the V BG spacing between the first and the second Coulomb peaks. The error bars come from the uncertainties in the Coulomb peak positions because of current noise. ( c ) Electron g -factors of the ground state for various V EDL . The error bars arise from errors both in the linear fit of the data in Fig. 5b (dashed line) and in the back-gate lever-arm factors (see Supplementary Fig. S6 ). ( d ) Schematic energy band diagram of the QD sample with negative V EDL (approximately −0.5 V). The conduction and the valence bands of the InAs surface are pushed up and, as a result, InAs surface is depleted. ( e ) Energy band diagram with positive V EDL (~0.1 V). The surface energy band is bent down and the surface depletion layer vanishes, resulting in a larger confinement size of electrons. The dashed lines are guides for eyes. Full size image In Figs 4 and 5c (see also Fig. 6a and Supplementary Fig. S8 ), each physical parameter exhibits saturation tendency at high negative V EDL , especially at V EDL <−0.5 V; this may be caused by the electric field screening by holes accumulated on the surface of the QD as schematically illustrated in Fig. 2b . Owing to the narrow band gap of InAs (~0.4 eV) and the extremely high electric field strength by EDL gating, EDL gate voltage of V EDL approximately −0.5 V is enough to accumulate holes around the tip region of the InAs QDs. Unfortunately, the accumulation of holes could not be detected by transport measurements because of a large spatial separation between the nano-gap metal electrodes and the surface hole accumulation region. 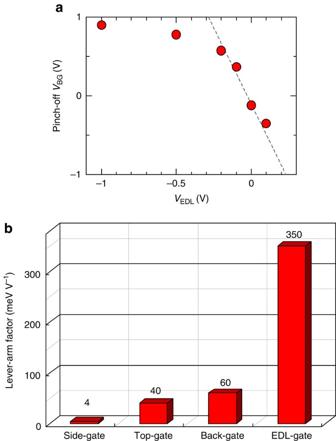Figure 6: Gating efficiency for various gating methods. (a) Pinch-off back-gate voltage,VBG, as a function ofVEDL. The dashed line is a guide for eyes. (b) Comparison of the lever-arm factors for various gating methods. The lever-arm factor is defined as the conversion ratio of the gate voltage to the shift in the energy levels. The lever-arm factor for the side gate was derived from Deaconet al.13and Kanaiet al.15The lever-arm factor for the back-gate was derived from this work (αBG~70 meV V−1) and Takahashiet al.14The lever-arm factor for the top-gate structure was derived fromSupplementary Fig. S9. The efficiency of EDL gating (350 meV V−1) is about 6, 9 and 90 times higher than that of the back gating (60 meV V−1), the top gating (40 meV V−1) and the side gating (4 meV V−1), respectively. In order to compare the lever-arm factors for different gating methods, we carefully chose the samples with almost the same nano-gap size (50 nm) and the QD location relative to the nano-gap electrodes (The QD is located at the centre of nano-gap metal electrodes as shown inFig. 1c). Figure 6: Gating efficiency for various gating methods. ( a ) Pinch-off back-gate voltage, V BG , as a function of V EDL . The dashed line is a guide for eyes. ( b ) Comparison of the lever-arm factors for various gating methods. The lever-arm factor is defined as the conversion ratio of the gate voltage to the shift in the energy levels. The lever-arm factor for the side gate was derived from Deacon et al . [13] and Kanai et al . [15] The lever-arm factor for the back-gate was derived from this work ( α BG ~70 meV V −1 ) and Takahashi et al . [14] The lever-arm factor for the top-gate structure was derived from Supplementary Fig. S9 . The efficiency of EDL gating (350 meV V −1 ) is about 6, 9 and 90 times higher than that of the back gating (60 meV V −1 ), the top gating (40 meV V −1 ) and the side gating (4 meV V −1 ), respectively. In order to compare the lever-arm factors for different gating methods, we carefully chose the samples with almost the same nano-gap size (50 nm) and the QD location relative to the nano-gap electrodes (The QD is located at the centre of nano-gap metal electrodes as shown in Fig. 1c ). Full size image Finally, in order to carefully compare the strength of the field effect of EDL gating on InAs QDs with that of conventional solid-gating methods, the lever-arm factors are used as the compared references. For a fair comparison, we consider only the voltage range of −0.1 V< V EDL <0.2 V, where screening by the surface charges is negligible. In Fig. 6a , the pinch-off back-gate voltage of the fabricated QD EDL transistor is plotted as a function of V EDL . The pinch-off V BG of the samples, which is defined as the V BG at which the first Coulomb conductance peak appears, strongly depends on V EDL and gradually increases as V EDL is reduced. The pinch-off V BG shifts from V BG =0.5 V to less than −1 V when V EDL is increased from −0.1 to 0.2 V. The total shift of >1.5 V in the pinch-off V BG corresponds to the energy shift of >105 meV by using the lever-arm factor α BG ~70 meV V −1 defined as the conversion ratio of V BG into energy for this sample ( Supplementary Fig. S6 ). The lever-arm factor for the EDL gating, α EDL , defined as the conversion ratio of V EDL into energy, can be calculated by dividing this energy shift of >105 meV by the EDL-gate voltage change Δ V EDL =0.3 V and determined to be α EDL >350 meV V −1 . Figure 6b shows the comparison of the lever-arm factors for various gating methods (see also Supplementary Fig. S9 ). Surprisingly, the efficiency of the EDL gating is 6–90 times higher than that observed in the conventional solid-gating techniques. This extremely high electric field strength by EDL gating will be very useful for electrical tuning of Rashba spin–orbit interaction [32] . Furthermore, the use of optically transparent ionic liquids as the gate dielectrics ( Fig. 1b ) potentially allows us to optically manipulate single-electron charge/spin states in QDs [6] , which is in clear contrast with the conventional metal top-gate structures, which block incoming light and hinder optical manipulation [33] . In summary, we have demonstrated the modulation of electron tunnelling in liquid-gated EDL transistor based on a single InAs QD coupled to nano-gap metal electrodes. The transport characteristics are dramatically modulated by the small EDL-gate voltage applied between the EDL-gate electrode and the InAs QD. The efficiency of gating is 6–90 times higher in the EDL gating than that in the conventional solid gating. The observed field effects can be explained by the change of the surface depletion thickness of InAs QDs, resulting in the change in the confinement potential in the QD. These results are the first demonstration of liquid-gated EDL transistors based on semiconductor QDs. The ability to electrically tune the quantum mechanical states of extremely small 0D nanostructures over a wide range potentially opens a way for their applications to quantum information technology. Sample preparation Self-assembled InAs QDs were grown by molecular beam epitaxy on a Si-doped (100)-oriented GaAs substrate. After successively growing a 100-nm-thick Si-doped GaAs layer and a 100-nm-thick undoped GaAs buffer layer, self-assembled InAs QDs were grown at 490 °C. A pair of Ti (5 nm)/Au (15 nm) electrodes separated by a 50-nm-wide gap were directly placed on an InAs QD and used as the source/drain electrodes. The metallurgical size of InAs QD used in this study was about 70 nm × 110 nm × 25 nm ( Fig. 1c ). In order to tune the electronic states in the InAs QDs, we fabricated a double-gate structure—that is, a liquid EDL gate and a degenerately Si-doped GaAs back-gate ( Fig. 1a ). Note that the EDL-gate electrode was used to accumulate or deplete charge carrier over a wide range, whereas the back-gate electrode was used for fine tuning of the discrete energy levels of the QD at low temperatures. The EDL-gate electrode was designed to be large enough to increase the electric field applied to QDs and formed directly on the GaAs layer ( Fig. 1a ). After bonding Au wires on the nano-gap source/drain electrodes, the EDL-gate electrodes and the back-gate electrodes, both the channel and the EDL-gate electrode were immersed in a small drop of ionic liquid to form a typical liquid-gated EDL transistor ( Fig. 1a,b ). The ionic liquid N , N -diethyl- N -(2-methoxyethyl)- N -methylammonium bis-(trifluoromethylsulfonyl)-imide (DEME-TFSI, from Kanto Chemical Co.) was used as the gate dielectric, and the bias voltage was applied between the EDL-gate electrode and the source electrodes, as shown in Fig. 1a . In order to avoid any possible interfacial electrochemistry between the ionic liquid and the InAs channel, transport measurements were mainly performed at 215 K and below, where it has been proved that the interfacial chemistry is suppressed by cooling [34] . Determination of the number of electrons in QD The sample presented in this study consists of a relatively large QD (the size is ~70 nm × 110 nm × 25 nm). Although the electrical contact to such a large QD is easy, there might be a possibility that the self-assembled QD is not single domain. In our case, we found that the major transport takes place only through one of the domains, even though the conduction through other domains may exist in parallel. In Supplementary Fig. S10 , we can see a slope that is very different from those of the diamonds (white dashed line). We ignored this parallel QD component and concentrated on the main transport channel. In Supplementary Fig. S10 , we cannot detect any signal at V BG less than −0.1 V within the current noise level of ~10 fA. Therefore, we identified this V BG region ( V BG less than −0.1 V) as N =0. In this large QD sample, influence of the parallel QD channel might become larger with the increase in the sample conductance (that is, with the increase in V EDL and/or N ), which may be the reason for blurred Coulomb diamonds for N ≥3. Determination of the charge addition energies In Fig. 3 , all the Coulomb stability diagrams were shown in the same colour scale to show that the conductance increases with increasing V EDL . However, such a plot is not suitable for determining the size of the Coulomb diamonds. Here we plot the same experimental results for N =1 Coulomb diamond in different colour scales in Supplementary Fig. S4 . The colour scales are chosen so that the boundary of the Coulomb diamond for N =1 can be determined more precisely. The size of N =1 Coulomb diamond becomes smaller with the increase in V EDL . Figures used to determine the boundary of the Coulomb diamond for N =2 are shown in Supplementary Fig. S5 . In single-electron transistors using InAs QDs, it is known that the single-electron tunnelling behaviour does not deviate far from the constant-interaction model. The deviation is typically <20% even in the few electron regime [11] , [12] , which appears as different slopes of the boundary lines of the Coulomb diamonds. Therefore, we determined the dashed lines in Supplementary Fig. S5 so that the boundary of the Coulomb diamond with positive and negative slopes becomes almost parallel with each other. The charge addition energy for N =2, E add (2), was determined by using these dashed lines. When the charge addition energy was polarity-dependent, the size of the Coulomb diamonds was determined as the average of the two. These figures show a clear tendency that the charge addition energy for N =2 becomes smaller with the increase in V EDL . The results on Δ E , defined as Δ E = E add (2)− E add (1), changes correspondingly as shown in Fig. 4c . On the other hand, we may observe a contribution of a parallel QD channel, particularly in the negative V SD region of the N =2 Coulomb diamonds in Supplementary Fig. S5 ; only the boundary shown by the black dashed lines has a slope that is very different from the white dashed lines, most likely because of the contribution of a parallel QD. Therefore, we should admit that the uncertainty in the size of N =2 Coulomb diamond is not small. However, even when we compare only the positive V SD region, the evolution of the Coulomb diamond size is clear and our claims are still solid. Determination of the lever-arm factor for top-gate structures We derived the lever-arm factor for the top-gate structures described in Fig. 6b . In order to compare the lever-arm factors for various gating methods, we carefully chose a sample with almost the same nano-gap size and the QD location relative to the nano-gap electrodes as those in Fig. 1c . A scanning electron microscope image of the QD sample for the top-gate is shown in Supplementary Fig. S9a . The nano-gap size is ~50 nm and the size of the QD is 120 nm × 80 nm × 25 nm. The QD is located at the centre of the nano-gap metal electrodes. These conditions are almost the same as those in the QD sample shown in Fig. 1c . The top-gate electrode was formed on top of the nano-gap electrodes by depositing a 25-nm HfO 2 thin film by atomic layer deposition and subsequently depositing a Ti/Au layer as schematically shown in Supplementary Fig. S9b . Supplementary Fig. S9c shows the Coulomb stability diagram obtained by measuring the differential conductance, d I /d V SD , as a function of the source-drain voltage, V SD , and the top-gate voltage, V TG , measured at 4.2 K. Coulomb diamonds are clearly observed. From the Coulomb diamonds, the lever-arm factor for the top-gate structures, α TG =Δ V SD /Δ V TG , was determined to be α TG ~40 meV/V. We checked one more sample with a top-gate structure and almost the same lever-arm factor was obtained. How to cite this article: Shibata, K. et al . Large modulation of zero-dimensional electronic states in quantum dots by electric-double-layer gating. Nat. Commun. 4:2664 doi: 10.1038/ncomms3664 (2013).